Sir2a regulates rDNA transcription and multiplication rate in the human malaria parasitePlasmodium falciparum The Plasmodium falciparum histone deacetylase Sir2a localizes at telomeric regions where it contributes to epigenetic silencing of clonally variant virulence genes. Apart from telomeres, PfSir2a also accumulates in the nucleolus, which harbours the developmentally regulated ribosomal RNA genes. Here we investigate the nucleolar function of PfSir2a and demonstrate that PfSir2a fine-tunes ribosomal RNA gene transcription. Using a parasite line in which PfSir2a has been disrupted, we observe that histones near the transcription start sites of all ribosomal RNA genes are hyperacetylated and that transcription of ribosomal RNA genes is upregulated. Complementation of the PfSir2a -disrupted parasites restores the ribosomal RNA levels, whereas PfSir2a overexpression in wild-type parasites decreases ribosomal RNA synthesis. Furthermore, we observe that PfSir2a modulation of ribosomal RNA synthesis is linked to an altered number of daughter merozoites and the parasite multiplication rate. These findings provide new insights into an epigenetic mechanism that controls malaria parasite proliferation and virulence. Malaria is caused by intracellular parasites of the genus Plasmodium that grow exponentially inside of human erythrocytes. Parasite intraerythrocytic development proceeds through well-defined stages (termed as ring, throphozoite and schizont) to generate up to 32 new parasites (named merozoites), which are released in the bloodstream to invade other erythrocytes. In Plasmodium falciparum , the species that causes the most severe form of the disease, this asexual cycle of multiplication takes 48 h to be completed. There is a poor understanding of the factors that cause severe malaria, although host and parasite genetic background, and environmental determinants are thought to have a crucial role [1] . The parasite multiplication rate (PMR) has been linked to severity of disease in rodent malaria studies [2] , [3] , [4] and in human P. falciparum [5] , [6] . In the case of rodent malaria Plasmodium yoelii , the erythrocyte binding ligand PyEBL was identified is a key component that controls growth rate [3] , the underlying mechanisms in P. falciparum remain poorly understood. The synthesis of eukaryotic ribosomal RNA (rRNA) determines ribosome production and the potential for cell growth and proliferation [7] . As in other eukaryotes, Plasmodium rRNA genes comprise the 18S–5.8S–28S genes that are transcribed by RNA Polymerase I (Pol I), but in a stage-specific manner. In the intraerythrocytic stages only two members of the unusual small rRNA gene family are actively transcribed ( A1 and A2 genes), whereas the others ( S1 and S2 genes) are predominantly transcribed when the parasite is in its mosquito vector [8] , [9] , [10] . To date, little is known about how this differential transcription is achieved and how the parasite regulates rRNA transcript levels in the different developmental life cycle stages. One candidate molecule to regulate Plasmodium rDNA transcription is the highly conserved NAD-dependent deacetylase Sir2, so-called sirtuin. The Plasmodium homologue of Sir2, PfSir2a, is the first identified epigenetic factor shown to be involved in transcriptional control of antigenic variation ( var gene family) in P. falciparum [11] , [12] , [13] . Like yeast Sir2, PfSir2a removes acetyl groups from the N-terminal tails of H3 and H4 in vitro in a NAD + -dependent manner [14] , it is associated with the telomeric clusters and also highly enriched in the nucleolus, the nuclear compartment dedicated to Pol I rDNA transcription [12] , [15] . However, so far no nucleolar function had been assigned to PfSir2a. The Sir2 family of deacetylases has a wide range of cellular targets, including the rDNA locus, where it controls transcription and rDNA stability. In yeast and African trypanosomes, Sir2 represses the transcription of genes artificially inserted within the repetitive rDNA [16] , [17] , [18] . In mammals, however, sirtuins can either repress [19] , [20] or activate [21] , [22] rDNA Pol I transcription. In addition, in yeast, Sir2 is known to prevent homologous recombination in the rDNA and the formation of toxic extrachromosomal circles [23] , [24] . In this study, we investigated the function of Sir2 at the atypical rDNA locus of the malaria parasite P. falciparum . Using mutant parasites, we demonstrate that transcription of the rRNA genes is modulated by PfSir2a at temperatures normally found in the human (37 °C) and mosquito (26 °C) hosts, resulting in changes in the number of merozoites produced in each cycle and consequently in the PMR. Our findings are highly relevant for changes in the host that cause a shift in the parasite’s NAD + /NADH ratio. Altering the silencing activity of PfSir2a could modify epigenetically the parasite’s intrinsic virulence and multiplication capacity. PfSir2a is a negative regulator of rDNA transcription In order to study the nucleolar function of PfSir2a during the parasite’s intraerythrocytic growth phase, we initially investigated the association of PfSir2a with the rDNA locus by using chromatin immunoprecipitation (ChIP). We observed a significant enrichment of PfSir2a at the rDNA locus, comparable to the previously reported at subtelomeric regions [12] ( Supplementary Fig. S1 ; P <0.05, Mann-Whitney (M-W) test). We next used a parasite line in which PfSir2a has been disrupted [11] and performed ChIP analysis of the acetylated histone H3 at lysine 9 (H3K9ac) distribution at the rDNA locus. H3K9ac is a known histone mark of Plasmodium active transcription [25] , [26] and one of the PfSir2a targets [14] , [27] . We observed an increase in H3K9ac levels downstream of the transcriptional initiation site of the active and silent rRNA genes ( A1 , A2 and S1 , S2 ; Fig. 1a ). Consistent with this increase in acetylation levels, we observed a 3-fold upregulation of the A- and S-type pre-rRNA transcripts in PfSir2a -disrupted parasites relative to wild-type parasites ( Fig. 1c ; P <0.05, M-W test). Importantly, the mature 18S rRNA levels ( Supplementary Fig. S2 ; P <0.05, M-W test), as well as the number of individual cytoplasmic ribosomes ( Fig. 1d ; P <0.0001, M-W test), were significantly increased in the mutant parasites, thus excluding a possible defect on rRNA maturation that could lead to an accumulation of pre-rRNA transcripts. We also confirmed that the copy number of rRNA genes was unchanged in the these mutant parasites ( Supplementary Fig. S3 ). Altogether, these results establish PfSir2a as a negative regulator of rRNA gene transcription in P. falciparum intraerythrocytic stages. 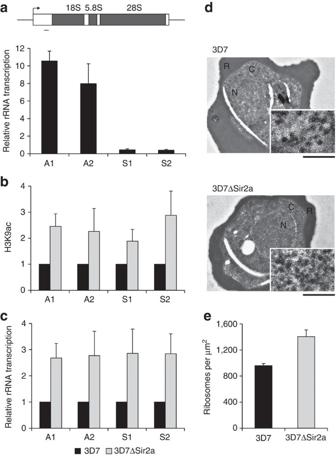Figure 1: PfSir2a is a negative regulator of rDNA transcription. (a) Schematic of aP. falciparumrRNA gene unit. It consists of a ~9 kb transcribed region coding for a 45S rRNA precursor, which is processed to mature 18S, 5.8S and 28S rRNAs. The parasite has four rDNA unit types, which are different in sequence, physically separated in the genome, and differentially transcribed over the developmental cycle. The graph shows the rRNA transcriptional profile in parasites synchronized on ring-stage, the stage at which Pol I transcription is greatest29(mean±s.e.m.,n=4). The arrow indicates the transcription start site and the direction of transcription. The bar indicates the position of the primers used for transcript and ChIP analysis. These primers independently detect the pre-rRNA transcripts from the four rRNA genes types (A1,A2,S1andS2). (b) Fold enrichment of H3K9ac on the individual rRNA genes obtained by ChIP analysis ofPfSir2a-disrupted parasites (3D7ΔSir2a, grey) relative to wild-type parasites (3D7, black) (mean±s.e.m.,n=3). (c) Relative transcription of the four rRNA genes in 3D7ΔSir2aparasites (grey) compared with the wild-type parasites (black) (mean±s.e.m.,n=4,P<0.05). (d) Representative sections of the ultrastructure from trophozoite stages of wild-type (3D7) and 3D7ΔSir2aparasites. The inset depicts the cytoplasmic ribosomal content. Scale bar, 1 μm in the main figure and 100 nm in the inset. R, red blood cell; C, parasite cytoplasm; N, parasite nucleus. (e) Quantification of the ribosomal content (mean±s.d.,n=2,P<0.0001). At least 20 cells were analysed for each of the two independent parasite preparations. Figure 1: PfSir2a is a negative regulator of rDNA transcription. ( a ) Schematic of a P. falciparum rRNA gene unit. It consists of a ~9 kb transcribed region coding for a 45S rRNA precursor, which is processed to mature 18S, 5.8S and 28S rRNAs. The parasite has four rDNA unit types, which are different in sequence, physically separated in the genome, and differentially transcribed over the developmental cycle. The graph shows the rRNA transcriptional profile in parasites synchronized on ring-stage, the stage at which Pol I transcription is greatest [29] (mean±s.e.m., n =4). The arrow indicates the transcription start site and the direction of transcription. The bar indicates the position of the primers used for transcript and ChIP analysis. These primers independently detect the pre-rRNA transcripts from the four rRNA genes types ( A1 , A2 , S1 and S2 ). ( b ) Fold enrichment of H3K9ac on the individual rRNA genes obtained by ChIP analysis of PfSir2a -disrupted parasites (3D7Δ Sir2a , grey) relative to wild-type parasites (3D7, black) (mean±s.e.m., n =3). ( c ) Relative transcription of the four rRNA genes in 3D7Δ Sir2a parasites (grey) compared with the wild-type parasites (black) (mean±s.e.m., n =4, P <0.05). ( d ) Representative sections of the ultrastructure from trophozoite stages of wild-type (3D7) and 3D7Δ Sir2a parasites. The inset depicts the cytoplasmic ribosomal content. Scale bar, 1 μm in the main figure and 100 nm in the inset. R, red blood cell; C, parasite cytoplasm; N, parasite nucleus. ( e ) Quantification of the ribosomal content (mean±s.d., n =2, P <0.0001). At least 20 cells were analysed for each of the two independent parasite preparations. Full size image To test whether PfSir2a may also control Pol I rDNA transcription in other parasite developmental stages, we compared the pre-rRNA levels in wild-type and PfSir2a -disrupted parasites subjected to 26 °C (temperature of the mosquito host) for ~6 h. Plasmodium rRNA gene transcription is known to be influenced by temperature [10] . As previously reported, we observed an upregulation of the S-type genes on both parasite populations. However, in the PfSir2a -disrupted parasites the levels of pre-rRNA transcripts were two times the level found in 3D7 wild-type parasites ( Supplementary Fig. S4 ). In conclusion, these results suggest a general PfSir2a transcriptional effect at the rDNA locus that may also be relevant during the insect stages of the parasite life cycle. PfSir2a disruption increases intraerythrocytic growth rate To assess the impact of the increase in rRNA levels and the number of ribosomes on parasite growth and proliferation, we monitored the progression of parasitemia (% of infected erythrocytes) of PfSir2a -disrupted parasites in parallel with that of wild-type. Starting from the same parasitemia, PfSir2a -disrupted parasites produced reproducibly significantly higher parasitemia than wild-type parasites (2–3-fold increase after three cycles, P <0.01, Wilcoxon test; Fig. 2a ). These data show for the first time a link between rRNA gene transcription and Plasmodium growth rate. We further addressed the question if the increased multiplication rate is due to a shortened asexual blood-stage cycle or due to higher number of daughter merozoites generated per erythrocytic schizont. Wild-type and the mutant parasites maintained a similar parasite asexual cycle duration (47.74±1.2 and 45.96±0.9 h for 3D7 and 3D7Δ Sir2a , respectively, P =0.2, M-W test; Fig. 2b ). However, the average number of merozoites did increase in the PfSir2a mutant parasite line (22.2±3.1 versus 18.8±3.1 in the wild-type, P <0.001, M-W test; Fig. 2c ). 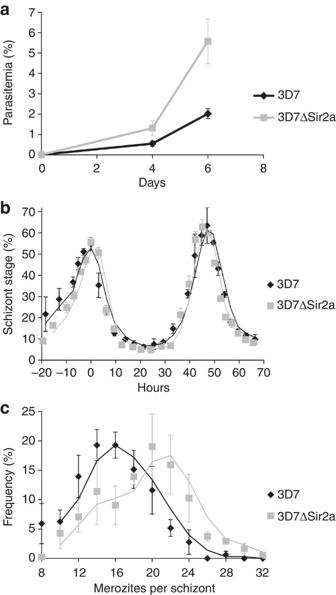Figure 2: PfSir2a disruption increases parasite intraerythrocytic growth rate. (a) Growth rate of the 3D7ΔSir2aparasites (grey squares) compared with that of wild-type 3D7 (black diamonds). The parasitemia (% of infected erythrocytes) on day 0 was set at 0.01% for both parasite lines and followed for three cycles (mean±s.e.m.,n=4,P<0.01). (b) Representative time course of 3D7 (black) and 3D7ΔSir2aparasite (grey) blood-stage cycles. The cycle time is the distance between the two peaks of schizonts; zero time corresponds to the first peak of mature schizonts. The average cycle duration for 3D7 and 3D7ΔSir2awas 47.74±1.2 and 45.96±0.9 h, respectively, (mean±s.d.,n=3,P=0.2). (c) Frequency distribution of the number of merozoites formed after schizogony in populations of wild-type 3D7 (black) and 3D7ΔSir2aparasites (grey) (mean±s.e.m.,n=5,P<0.001). Approximately 50–60 mature schizonts with clear separated merozoites and a single pigmented digestive vacuole were counted for each of the five independent experiments. Figure 2: PfSir2a disruption increases parasite intraerythrocytic growth rate. ( a ) Growth rate of the 3D7Δ Sir2a parasites (grey squares) compared with that of wild-type 3D7 (black diamonds). The parasitemia (% of infected erythrocytes) on day 0 was set at 0.01% for both parasite lines and followed for three cycles (mean±s.e.m., n =4, P <0.01). ( b ) Representative time course of 3D7 (black) and 3D7Δ Sir2a parasite (grey) blood-stage cycles. The cycle time is the distance between the two peaks of schizonts; zero time corresponds to the first peak of mature schizonts. The average cycle duration for 3D7 and 3D7Δ Sir2a was 47.74±1.2 and 45.96±0.9 h, respectively, (mean±s.d., n =3, P =0.2). ( c ) Frequency distribution of the number of merozoites formed after schizogony in populations of wild-type 3D7 (black) and 3D7Δ Sir2a parasites (grey) (mean±s.e.m., n =5, P <0.001). Approximately 50–60 mature schizonts with clear separated merozoites and a single pigmented digestive vacuole were counted for each of the five independent experiments. Full size image Complementation of the PfSir2a disruption To confirm the observed phenotypic changes in the PfSir2a -disrupted parasites that were due to the absence of a functional PfSir2a, we generated complemented parasites that express PfSir2a from an episome. PfSir2a was fused to the red fluorescent protein mCherry and expression directed by a constitutively active promoter (calmodulin) ( Fig. 3a ). PfSir2a::mCherry was enriched at the nuclear periphery, forming foci that resemble the perinuclear pattern (telomeric clusters and nucleolus) previously shown for the native PfSir2a ( Fig. 3b ) [12] , [15] . Importantly, complementation of the PfSir2a disruption restored the pre-rRNA transcript levels for A- and S-types ( Fig. 3c ), and displayed a growth rate and merozoite numbers similar to that of the wild-type parasites ( Fig. 4a , Table 1 ). PfSir2a -disrupted parasites transfected with the control plasmid did not exhibit significant differences in the multiplication rate ( P =0.42, M-W test) or in merozoite formation ( P =0.49, M-W test), confirming that the observed changes in PfSir2a -disrupted parasites are indeed mediated by PfSir2a ( Table 1 ). 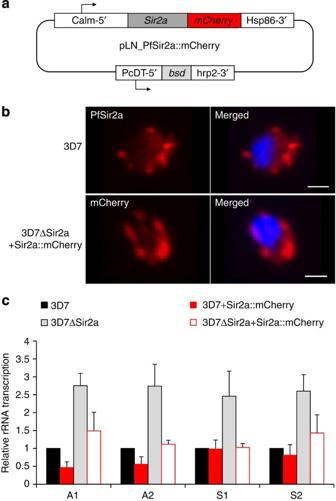Figure 3: Complementation of 3D7ΔSir2aand PfSir2a overexpression. (a) Schematic of the plasmid used for PfSir2a episomal expression (pLN_PfSir2a::mCherry). The arrow indicates the direction of transcription. (b) Immunofluorescence assay in paraformaldehyde fixed ring-stage parasites with anti-PfSir2a antibodies (red) in wild-type parasites (first row) and anti-mCherry antibodies (red) in 3D7ΔSir2a+Sir2a::mCherry parasites (second row). Nuclei of ring-stage parasites were stained with Dapi (blue). Scale bar, 1 μm. (c) Relative transcription of individual rRNA genes in 3D7ΔSir2a(grey), complemented 3D7ΔSir2a(3D7ΔSir2a+Sir2a::mCherry; red line) and wild-type overexpressing Sir2a (3D7+Sir2a::mCherry; red) compared with the wild-type parasites (3D7; black) (mean±s.e.m.,n=3).Pvalues calculated relative to the wild-type 3D7 are as follows: 3D7ΔSir2a+Sir2a::mCherry, NS; 3D7ΔSir2a,P<0.05; 3D7+Sir2a::mCherry,P<0.05 for theA1rRNA gene. Figure 3: Complementation of 3D7Δ Sir2a and PfSir2a overexpression. ( a ) Schematic of the plasmid used for PfSir2a episomal expression (pLN_PfSir2a::mCherry). The arrow indicates the direction of transcription. ( b ) Immunofluorescence assay in paraformaldehyde fixed ring-stage parasites with anti-PfSir2a antibodies (red) in wild-type parasites (first row) and anti-mCherry antibodies (red) in 3D7Δ Sir2a +Sir2a::mCherry parasites (second row). Nuclei of ring-stage parasites were stained with Dapi (blue). Scale bar, 1 μm. ( c ) Relative transcription of individual rRNA genes in 3D7Δ Sir2a (grey), complemented 3D7Δ Sir2a (3D7Δ Sir2a +Sir2a::mCherry; red line) and wild-type overexpressing Sir2a (3D7+Sir2a::mCherry; red) compared with the wild-type parasites (3D7; black) (mean±s.e.m., n =3). P values calculated relative to the wild-type 3D7 are as follows: 3D7Δ Sir2a+Sir2a::mCherry , NS; 3D7Δ Sir2a , P <0.05; 3D7+ Sir2a::mCherry , P <0.05 for the A1 rRNA gene. 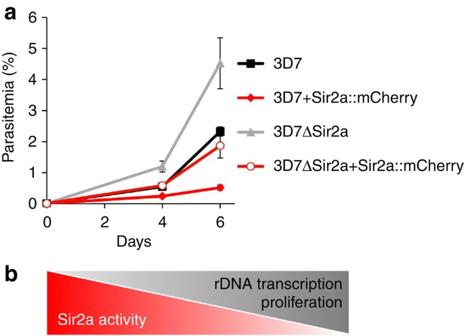Figure 4: Parasite multiplication rate altered with varying levels of PfSir2a. (a) Growth rate of the complemented 3D7ΔSir2a(open red circles) and PfSir2a overexpressing parasites (red diamonds) compared with that of 3D7ΔSir2a(grey triangles) and 3D7 (black squares) parasites. As inFig. 2b, the initial parasitemia was set at 0.01% for all parasite lines (mean±s.e.m.,n=5). A summary of the parasite multiplication rate after two cycles and the average number of merozoites per schizont (segmented stage) in the various transgenic parasite lines, including the transfection controls is shown inTable 1. (b) Schematic representation of the observed inverse correlation between the PfSir2a levels and the rDNA transcription and parasite proliferation. Our data predict that the lower is the PfSir2a silencing activity the higher is the rDNA transcription and parasite multiplication rates, and vice-versa. Full size image Figure 4: Parasite multiplication rate altered with varying levels of PfSir2a. ( a ) Growth rate of the complemented 3D7Δ Sir2a (open red circles) and PfSir2a overexpressing parasites (red diamonds) compared with that of 3D7Δ Sir2a (grey triangles) and 3D7 (black squares) parasites. As in Fig. 2b , the initial parasitemia was set at 0.01% for all parasite lines (mean±s.e.m., n =5). A summary of the parasite multiplication rate after two cycles and the average number of merozoites per schizont (segmented stage) in the various transgenic parasite lines, including the transfection controls is shown in Table 1 . ( b ) Schematic representation of the observed inverse correlation between the PfSir2a levels and the rDNA transcription and parasite proliferation. Our data predict that the lower is the PfSir2a silencing activity the higher is the rDNA transcription and parasite multiplication rates, and vice-versa. Full size image Table 1 PMR and merozoite numbers per schizont in the various transgenic parasite lines. Full size table PfSir2a overexpression in wild-type parasites To further verify the role of PfSir2a in repressing rRNA gene transcription and parasite growth, we transfected wild-type parasites with the same plasmid used for the complementation studies ( Fig. 3a ). As for the complemented parasites, we examined the resistant parasites by qRT–PCR to confirm the increase in PfSir2a transcript levels, and by microscopy to monitor the expression and localization of the PfSir2a::mCherry fusion protein (data not shown). The episomal PfSir2a overexpression in wild-type parasites resulted in significantly lower number of merozoites per schizont (12.3±2.8, P <0.0001, M-W test; Table 1 ), as well as lower levels of parasitemia than those of wild-type or the transfection control parasites ( P <0.0001 and P <0.001, respectively, M-W test; Fig. 4a , Table 1 ). In terms of rRNA synthesis, the transcript levels of A1 and A2 rRNA genes were approximately two-fold downregulated, whereas pre-rRNA transcript levels of S-types appeared unchanged ( Fig. 3c ), suggesting that in blood-stages the S-type rRNA genes are completely repressed. The Plasmodium Sir2 homologue PfSir2a has been of great interest because of its role in the epigenetic regulation of the var gene family, the most clinically relevant multicopy gene family, which encodes for the major surface antigen PfEMP1 [11] , [12] , [27] , [28] . Although the PfSir2a subcellular enrichment in the nucleolus has been reported earlier [12] , [15] its function in the rDNA biology remained unknown. Plasmodium rDNA has also received considerable attention, as it bears several features not found in other eukaryotes [8] , [9] , [10] . Because of its repetitive nature, the previous transcriptomic studies of PfSir2a -disrupted parasites excluded rDNA from the microarray chip [11] , [28] . In this work, we examined the rRNA by using primers that specifically detect the four individual rRNA gene types. In the PfSir2a mutant parasites, we observed a significant increase in all types of rRNA transcripts, associated with histone hyperacetylation. Thus, revealing a novel PfSir2a function as a regulator of rDNA chromatin structure, thereby exerting control of rRNA transcript levels. The possibility of PfSir2a having a role in preventing recombination among the few rDNA units clustered in the nucleolus [29] , as seen in yeast [23] , was also investigated. However, no apparent changes were detected in the rDNA restriction pattern (AS, manuscript in preparation), suggesting that other silencing/heterochromatic factors may be involved in controlling recombination in the nucleolus. It is remarkable that while Sir2 localization in the nucleolus appears evolutionary conserved, its function therein is quite divergent. Also divergent is the role of the second Plasmodium sirtuin, PfSir2b, a rather distant Sir2 homologue that appears to cooperate with PfSir2a to regulate virulence genes and antigenic variation [28] . PfSir2b -disrupted parasites do not show de-repression of rRNA genes nor effects on blood-stage proliferation and fitness ( Supplementary Fig. S5 ). The subcellular location of PfSir2b has not yet been reported. The increased levels of rRNA transcripts in the parasites lacking a functional PfSir2a resulted in higher numbers of individual cytoplasmic ribosomes and increased parasite proliferation. The fact that no significant transcriptional changes were observed for associated ribosomal proteins or translational factors [11] , [28] , supports the idea that in Plasmodium , like in other eukaryotes, ribosome production is limited by the transcription of the rDNA itself. The observed increased number of merozoites formed on each round of parasite multiplication in the PfSir2a mutant parasites suggests that higher ribosome numbers are likely to signal additional mitotic divisions to the parasite. Another possibility is that PfSir2a may directly interact with regulatory factors of parasite DNA synthesis and/or mitosis, as described for other sirtuins in mammals [30] . So far, the only known PfSir2a targets are the acetylated histones [12] , [14] and the recently identified PfAlba protein family [31] . It would be interesting to explore the PfSir2a interactome further. Like all members of the eukaryotic Sir2 family [32] , PfSir2a is dependent on NAD + for its deacetylase activity [14] . As NAD + is a metabolic cofactor, Sir2 proteins can be considered as sensors of the cell’s metabolic state [33] , [34] . Hence, it is possible that PfSir2a may act as a metabolic sensor molecule balancing the malaria parasite’s energy status with rRNA synthesis and parasite proliferation. Indeed, culturing of P. falciparum blood-stage parasites in low-glucose conditions has been associated to a decrease in rRNA transcript levels [35] . Likewise, glucose depletion in HeLa cells affects ribosome biogenesis, and the underlying mechanism involves a SIRT1 protein complex [19] . Thus, it is tempting to speculate that the hypoglycemia observed in patients with severe malaria [36] implicates PfSir2a to couple changing energy status with rDNA transcription and proliferation of blood-stage parasites. Apart from the metabolic changes on NAD + /NADH, there are other environmental factors likely to modulate PfSir2a activity. These may include high temperatures (>40 °C) found in malaria-induced febrile illness, which have been reported to increase PfSir2a transcript levels [37] and also to decrease transcription of Pf rDNA [10] . In conclusion, our data predict that lower/higher P. falciparum PfSir2a activity in malaria patients could establish epigenetically determined variable rDNA transcription and parasite proliferation rates in genetically identical parasites ( Fig. 4b ). This knowledge is highly relevant for clinical studies exploring the underlying mechanisms of malaria virulence. Parasite culture P. falciparum parasite lines were cultured in human O + erythrocytes at 4% haematocrit in RPMI 1640 supplemented with 0.5% Albumax II (Invitrogen), 200 μM Hypoxanthine and 20 μg ml −1 Gentamicin. Parasites were incubated at 37 or 26 °C in an atmosphere of 5% oxygen, 5% carbon dioxide and 90% nitrogen. Synchronization of cultures consisted of consecutive treatments with 5% Sorbitol (Sigma) and Plasmion (Laboratoire Fresenius Kabi). We estimated that the parasites were synchronized within a window of 4–6 h by Giemsa staining. Plasmids and parasite transfection A synthetic gene construct coding for PfSir2a fused with mCherry sequence was obtained (GeneArt) and cloned in frame into the backbone plasmid vector pLN_ENR_GFP [38] . The vector control was obtained by removing the Pfenr gene from the pLN_ENR_GFP [38] by enzymatic digestion. Ring-stage parasite lines 3D7 and 3D7Δ Sir2a were transfected with pLN_PfSir2a::mCherry and pLN_GFP plasmids by electroporation, and drug selected using 2.5 μg ml −1 of blasticidin hydrochloride (BSD). For 3D7 wild-type transfections, BSD-resistant parasites appeared after 5–7 weeks of culture. For the 3D7Δ Sir2a transfections, BSD-resistant parasites appeared 3–4 weeks of culture, after which a double selection was applied (2.5 μg ml −1 BSD and 2 μM pyrimethamine (PYR)). The presence of the plasmid and integrity of the insert were confirmed by PCR using different combinations of primers. Parasite growth rate analysis To assess the relative growth rate of 3D7 wild-type and transgenic parasite lines, we used highly synchronous 4% haematocrit cultures at 0.01% parasitemia. The culture medium was changed daily (without adding new erythrocytes). The medium for transgenic lines contained the following drugs: 3D7Δ Sir2a , 2 μM PYR; 3D7+ Sir2a :: mCherry and 3D7+vector, 2.5 μg ml −1 BSD; 3D7Δ Sir2a + Sir2a :: mCherry and 3D7Δ Sir2a +vector, 2.5 μg ml −1 BSD and 2 μM PYR. Samples were collected every 24 h for staining with Giemsa and/or the fluorescent DNA-specific dye SYBR Green I [39] , [40] . To determine parasitemia in the Giemsa-stained thin blood smears, images of 1,000–2,000 erythrocytes were randomly acquired and the percentage of infected erythrocytes counted semi-automatically using ImageJ ( http://rsbweb.nih.gov/ij/ ). This software was also used for counting of the number of merozoites per schizont on Giemsa-stained smears. The SYBR Green I stained samples were analysed on a CyFlow SL Blue (Partec) flow cytometer and the data evaluated using FlowJo software (TreeStar) to determine the percentage of infected erythrocytes. Parasite cycle duration analysis To determine cell-cycle length, we used highly synchronous 4% haematocrit cultures at 0.1% parasitemia. Fifty microlitre of culture was collected every 2–3 h and stained with SYBR Green I as above. The distribution of parasite stages of each sample was analysed by flow cytometry for DNA content. As defined previously [41] , the cycle time corresponds to the duration between two peaks of schizonts. To calculate the percentage of schizonts we gated on parasites showing N >4 ( N is the number of nuclei). The values were plotted against time and fitted to a sine wave function using GraphPad Prism software with the following equation: Y is the percentage of schizonts, X is the time, m 1 is the shift in the y axis, m 2 is the shift in the x axis and wavelength is the cycle length. Fluorescence microscopy Immunofluorescence assays were performed as previously described [15] in ring-stage parasites. Antibody dilutions were as follows: anti-PfSir2a, 1:100; anti-mCherry (Abcam, ab-62341), 1:5,000; and anti-rabbit highly cross-absorbed Alexa-Fluor-488-conjugated (Invitrogen), 1:500. Images were taken using a Nikon Eclipse 80i microscope with a CoolSnap HQ2 camera (Photometrics). NIS Elements 3.0 software (Nikon) was used for acquisition and ImageJ for composition. Electron microscopy Infected erythrocytes were fixed in 1% glutaraldehyde in RPMI-HEPES, and embedded in LR Gold resin (London Resin Company Ltd, UK) as previously described [42] . Ultrathin sections of 55 nm were collected, stained with 4% uranyl acetate and observed by using a JEOL JEM-1200EX electron microscope. Quantification of ribosomal content was performed as described [43] by manually counting of the number of ribosomes in defined areas of the cytoplasm (squares of 0.2 × 0.2 μm 2 ) using ImageJ. The average of at least three squares per parasite was calculated and expressed as ribosomes per square micrometre. Transcript analysis Total RNA was isolated using the Trizol method from ring-stage synchronized cultures (stage at which Pol I transcription is greatest [29] ). As rRNA gene transcription is very sensitive to temperature changes [10] , all the operations prior Trizol extraction were performed at 37 °C, except for experiments on Supplementary Fig. S4 , which were carried out at room temperature. Extracted RNA was DNAse treated, reverse transcribed and analysed by quantitative PCR (qPCR) using the set of primers designed in a previous work [29] . ΔΔCt analysis was used to calculate the relative expression of each rRNA gene, normalized to the geometric mean of three reference genes: PFB0295w, PF07_0073 and MAL8P1.151 ( www.plasmodb.org ). The selected three genes satisfy the following criteria: unchanged in the 3D7 versus 3D7Δ Sir2a [11] , unchanged over the 48 h cycle and expression in fair abundance. The sequence of primers is listed in Supplementary Table S1 . ChIP analysis The ChIP assay was performed in ring-stage synchronized parasites using a previously described protocol [26] . Immunoprecipitation was performed at 4 °C overnight with a 1:100 dilution of anti-H3K9ac (Upstate, 07-352). Immunoprecipitated DNA was analysed by qPCR, as described above. qPCR was also performed in dilutions of purified input DNA, to calculate the amount of target sequence in immunoprecipitated chromatin relative to the amount of target sequence in input (% of input). Statistical analysis Significance between the transgenic lines and 3D7 wild-type was calculated using the GraphPad Prism software, and is indicated as follows: not significant (NS) P ≥0.05; * P <0.05; ** P <0.01; *** P <0.001; **** P <0.0001. How to cite this article: Mancio-Silva, L. et al . Sir2a regulates rDNA transcription and multiplication rate in the human malaria parasite Plasmodium falciparum . Nat. Commun. 4:1530 doi: 10.1038/ncomms2539 (2013).